Tyr26 phosphorylation of PGAM1 provides a metabolic advantage to tumours by stabilizing the active conformation How oncogenic signalling coordinates glycolysis and anabolic biosynthesis in cancer cells remains unclear. We recently reported that the glycolytic enzyme phosphoglycerate mutase 1 (PGAM1) regulates anabolic biosynthesis by controlling intracellular levels of its substrate 3-phosphoglycerate and product 2-phosphoglycerate. Here we report a novel mechanism in which Y26 phosphorylation enhances PGAM1 activation through release of inhibitory E19 that blocks the active site, stabilising cofactor 2,3-bisphosphoglycerate binding and H11 phosphorylation. We also report the crystal structure of H11-phosphorylated PGAM1 and find that phospho-H11 activates PGAM1 at least in part by promoting substrate 3-phosphoglycerate binding. Moreover, Y26 phosphorylation of PGAM1 is common in human cancer cells and contributes to regulation of 3-phosphoglycerate and 2-phosphoglycerate levels, promoting cancer cell proliferation and tumour growth. As PGAM1 is a negative transcriptional target of TP53 , and is therefore commonly upregulated in human cancers, these findings suggest that Y26 phosphorylation represents an additional acute mechanism underlying phosphoglycerate mutase 1 upregulation. The Warburg effect describes the observation that tumour cells take up more glucose than normal tissue and favour glycolysis even in the presence of oxygen. This phenomenon is not limited to solid tumours, as leukaemia cells are also highly glycolytic [1] , [2] . One metabolic advantage of the Warburg effect is that a boost in aerobic glycolysis in tumour cells generates more ATP more quickly than normal cells that rely on oxidative phosphorylation [3] . Moreover, tumour cells use glycolytic intermediates for anabolic biosynthesis of macromolecules including nucleotides, amino acids and fatty acids, which are used to produce RNA/DNA, proteins and lipids, respectively. These ‘building blocks’ are necessary for cell proliferation, and their expeditive production is crucial to fulfill the demands of rapidly growing tumours [3] . However, how tumour cells coordinate glycolysis and anabolic biosynthesis remains largely unknown. We recently reported that the glycolytic enzyme phosphoglycerate mutase 1 (PGAM1) regulates anabolic biosynthesis by controlling intracellular levels of its substrate 3-phosphoglycerate (3-PG) and product 2-phosphoglycerate (2-PG) [4] . PGAM1 catalyses the conversion of 3-PG to 2-PG, a crucial step in glycolysis. PGAM1 is activated upon binding of the cofactor 2,3-bisphosphoglycerate (2,3-BPG), which phosphorylates PGAM1 at histidine 11 (H11) by transferring the C3 phosphate group to H11 (ref. 5 ). During the conversion of 3-PG to 2-PG by PGAM1, phospho-H11 of PGAM1 is positioned to facilitate transfer of phosphate from phospho-H11 to C-2 of the substrate 3-PG. This creates a 2,3-BPG intermediate in the catalytic pocket, which in turn ‘re-phosphorylates’ H11 by transferring the C3 phosphate group back to H11 to return the enzyme to its initial H11-phosphorylated, fully activated state and allow for release of product 2-PG. Such a ‘ping-pong’ mechanism of PGAM1 activation involving catalytic H11 phosphorylation by 2,3-BPG has been known for decades, and is supported by kinetic studies [6] , [7] and isolation of the phospho-H11 containing peptide [8] . However, the structural mechanisms underlying 2,3-BPG binding and how H11 phosphorylation activates PGAM1 remain unknown. PGAM1 activity has been reported to be upregulated in many cancers, including hepatocellular carcinoma and colorectal cancer [9] , [10] , probably due to increased PGAM1 gene expression resulting from loss of TP53 , as PGAM1 is a negative transcriptional target of TP53 (refs 11 , 12 , 13 ). In consonance with this, we found that PGAM1 protein expression and enzyme activity levels are upregulated in human primary leukaemia cells from diverse leukaemia patients with acute myeloid leukaemia, chronic myelogenous leukaemia and B-cell acute lymphoblastic leukaemia [4] . Moreover, we found that 3-PG binds to and inhibits 6-phosphogluconate dehydrogenase (6PGD) in the oxidative pentose phosphate pathway (PPP), while 2-PG activates 3-PG dehydrogenase (PHGDH) to provide feedback control of 3-PG levels. Inhibition of PGAM1 by shRNA or a small molecule inhibitor PGMI-004A results in increased 3-PG and decreased 2-PG levels in cancer cells, leading to significantly decreased glycolysis, PPP flux, biosynthesis, cell proliferation and tumour growth. Here, we report that Y26 phosphorylation of PGAM1 is common in human cancers, providing a proliferative advantage. Structural analyses revealed a novel mechanism in which Y26 phosphorylation enhances PGAM1 activation by stabilising the active conformation of PGAM1. We were also the first to crystalise H11-phosphorylated PGAM1 and structural analysis suggests that phospho-H11 activates PGAM1 at least in part by promoting substrate 3-PG binding. Thus, Y26 phosphorylation of PGAM1 represents a novel, acute mechanism underlying PGAM1 upregulation in cancer cells in addition to chronic changes regulated by TP53 . Y26 phosphorylation enhances 2,3-BPG-dependent PGAM1 activity Our phospho-proteomics studies identified PGAM1 as phosphorylated at multiple tyrosine sites including Y26, Y92, Y119 and Y133 in murine haematopoietic Ba/F3 cells expressing constitutively active ZNF198–FGFR1 fusion tyrosine kinase [14] ( Fig. 1a ). In consonance with this observation, GST-tagged PGAM1 was tyrosine phosphorylated in COS7 cells transiently co-transfected with plasmids encoding FGFR1 wild-type (WT), but not in cells co-expressing GST-PGAM1 and a kinase-dead form of FGFR1 ( Fig. 1b ). We further confirmed this in an in vitro kinase assay where active, recombinant FGFR1 (rFGFR1) or EGFR (rEGFR) directly phosphorylated purified, Flag-tagged recombinant PGAM1 (rPGAM1) at tyrosine residues ( Fig. 1c ). 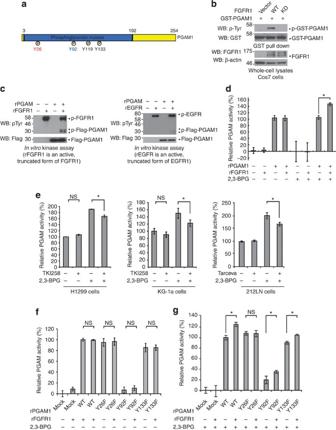Figure 1: Y26 phosphorylation enhances PGAM1 activity. (a) Schematic representation of PGAM1 with identified tyrosine phosphorylation sites in phospho-proteomics studies. (b) Immunoblotting of cell lysates for tyrosine phosphorylation of GST-PGAM1 when coexpressed with FGFR1 WT or a kinase-dead form (KD). (c) Active, rFGFR1 (left) and EGFR (rEGFR; right) were incubated with Flag-PGAM1 inin vitrokinase assays. Tyrosine phosphorylation of Flag-PGAM1 was assessed by western blot. (d) Enzyme activity of recombinant PGAM1 (rPGAM1) treated with or without rFGFR1 was measured in the presence or absence of 10 μM 2,3-BPG. (e) PGAM1 activity in the presence or absence of 2,3-BPG in cell lysates from human lung cancer H1299 (left) and leukaemia KG-1a cells (middle) treated with FGFR1 inhibitor TKI258, or head and neck cancer 212LN cells (right) treated with EGFR inhibitor Tarceva. (f–g) Activity of diverse PGAM1 Y→F mutants treated with FGFR1 in the presence (g) or absence (f) of 10 μM 2,3-BPG. The values were normalised to the activity level of WT PGAM1 without FGFR1 treatment. The error bars represent mean values±s.d. from three independent experiments (*0.01<P<0.05; **P<0.01). Figure 1: Y26 phosphorylation enhances PGAM1 activity. ( a ) Schematic representation of PGAM1 with identified tyrosine phosphorylation sites in phospho-proteomics studies. ( b ) Immunoblotting of cell lysates for tyrosine phosphorylation of GST-PGAM1 when coexpressed with FGFR1 WT or a kinase-dead form (KD). ( c ) Active, rFGFR1 (left) and EGFR (rEGFR; right) were incubated with Flag-PGAM1 in in vitro kinase assays. Tyrosine phosphorylation of Flag-PGAM1 was assessed by western blot. ( d ) Enzyme activity of recombinant PGAM1 (rPGAM1) treated with or without rFGFR1 was measured in the presence or absence of 10 μM 2,3-BPG. ( e ) PGAM1 activity in the presence or absence of 2,3-BPG in cell lysates from human lung cancer H1299 (left) and leukaemia KG-1a cells (middle) treated with FGFR1 inhibitor TKI258, or head and neck cancer 212LN cells (right) treated with EGFR inhibitor Tarceva. ( f – g ) Activity of diverse PGAM1 Y→F mutants treated with FGFR1 in the presence ( g ) or absence ( f ) of 10 μM 2,3-BPG. The values were normalised to the activity level of WT PGAM1 without FGFR1 treatment. The error bars represent mean values±s.d. from three independent experiments (*0.01< P <0.05; ** P <0.01). Full size image PGAM1 is believed to be activated upon binding of cofactor 2,3-BPG, which was suggested to ‘phosphorylate’ PGAM1 at histidine 11 (H11) by transferring the C3 phosphate to H11 (ref. 5 ). In a PGAM1 enzyme assay coupled with the FGFR1 in vitro kinase assay, we found that rFGFR1 significantly enhanced rPGAM1 enzyme activity only in the presence but not absence of 2,3-BPG ( Fig. 1d ). Notably, purified PGAM1 in the absence of 2,3-BPG shows comparable level of enzyme activity as PGAM1 in the presence of 2,3-BPG, indicating that the purified recombinant PGAM1 is H11-phosphorylated and activated to a certain extent, which may be due to modification from bacteria or 3-PG applied in the experiments contaminated with 2,3-BPG as previously described [15] . Nevertheless, these data suggest that FGFR1-dependent tyrosine phosphorylation ‘further’ enhances PGAM1 activation. In addition, in a PGAM1 enzyme activity assay, incubation with cofactor 2,3-BPG significantly activates PGAM1 in cell lysates from FGFR1-expressing lung cancer H1299 and leukaemia KG-1a cells ( Fig. 1e ; left and middle, respectively) and EGFR-expressing head and neck cancer 212LN cells ( Fig. 1e ; right), while treatment with the FGFR1 small molecule inhibitor TKI258 or EGFR inhibitor Tarceva significantly decreases PGAM1 enzyme activity, only in the presence but not absence of 2,3-BPG in H1299 and KG-1a or 212LN cells, respectively. We next performed mutational analysis and found that, in the absence of 2,3-BPG, tyrosine phosphorylation by FGFR1 did not alter enzyme activity of rPGAM1 WT, Y26F or Y133F. Interestingly, Y92F mutant lost PGAM1 enzyme activity in the presence and absence of rFGFR1, suggesting that Y92 is intrinsically required for PGAM1 enzyme activity ( Fig. 1f ). In contrast, in the presence of 2,3-BPG, rFGFR1 significantly activates rPGAM1 WT and Y133F mutant ( Fig. 1g ). However, substitution of Y26 abolished the FGFR1-dependent increase in the PGAM1 enzyme activity. Y92F mutant again showed a very low level of PGAM1 activity, however, incubation with rFGFR1 resulted in significantly increased PGAM1 enzyme activity of Y92F in the presence of 2,3-BPG ( Fig. 1g ). These data together suggest that Y26 phosphorylation is responsible for mediating FGFR1-dependent, ‘enhanced’ activation of PGAM1 in the presence of 2,3-BPG. Y26 phosphorylation PGAM1 enhances H11 phosphorylation Structural studies revealed that both H11 and Y92 are directly proximal to the active site where both cofactor (2,3-BPG) and substrate (3-PG) bind ( Fig. 2a ) [16] , suggesting that Y92 may be crucial for 2,3-BPG binding and PGAM1 activity, consistent with our observation that substitution of Y92 abolishes PGAM1 enzyme activity ( Fig. 1f ). This is also consistent with a previous report that S14, T23, G24, R90, Y92, K99, R116 and R117 are involved in binding of cofactor 2,3-BPG and substrate 3-PG, which share the same binding pocket on PGAM1 (ref. 17 ). Y26 is also close to the catalytic site ( Fig. 2a ); as Y26-phoshorylation by FGFR1 enhances PGAM1 in the presence of 2,3-BPG, this suggests a potential mechanism wherein Y26 phosphorylation by FGFR1 may stabilise the H11-phosphorylated PGAM1. 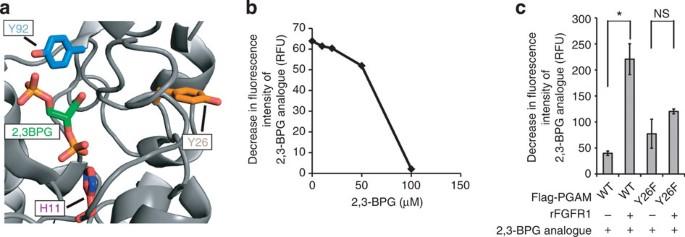Figure 2: Y26 phosphorylation promotes cofactor 2,3-BPG binding to PGAM1. (a) Cartoon representation of 2,3-BPG location from structure 3FDZ superposed on PGAM1 (PDB accession code: 1YFK). H11 and Y92 are directly proximal to and Y26 is also close to cofactor (2,3-BPG)/substrate (3-PG) binding site. (b) 2,3-BPG analogue (8-hydroxy-1,3,6-pyrenetrisulfonate) competes with 2,3-BPG for binding to rPGAM1 protein, where 3 μM 2,3-BPG analogue was mixed with different concentrations of 2,3-BPG in reaction mixture containing 100 mM Tris-HCl (pH 7.5). Fluorescence intensity of 2,3-BPG analogue (ex: 362 nm, em: 520 nm) was measured before and 5 min after the addition of 2.3 μM rPGAM1 protein to the reaction mixture. Decrease in fluorescence intensity of 2,3-BPG analogue indicates 2,3-BPG analogue binding to rPGAM1 protein. The values are presented as relative fluorescence units (RFU). (c) Purified Flag-PGAM1 WT or Y26F were incubated with cofactor (represented by 2,3-BPG analogue, 8-hydroxy-1,3,6-pyrenetrisulfonate). The cofactor binding affinity was determined by decrease in fluorescence intensity of the analogue. The values are presented as RFU. The error bars represent mean values±s.d. from three independent experiments (*0.01<P<0.05; **P<0.01). Figure 2: Y26 phosphorylation promotes cofactor 2,3-BPG binding to PGAM1. ( a ) Cartoon representation of 2,3-BPG location from structure 3FDZ superposed on PGAM1 (PDB accession code: 1YFK). H11 and Y92 are directly proximal to and Y26 is also close to cofactor (2,3-BPG)/substrate (3-PG) binding site. ( b ) 2,3-BPG analogue (8-hydroxy-1,3,6-pyrenetrisulfonate) competes with 2,3-BPG for binding to rPGAM1 protein, where 3 μM 2,3-BPG analogue was mixed with different concentrations of 2,3-BPG in reaction mixture containing 100 mM Tris-HCl (pH 7.5). Fluorescence intensity of 2,3-BPG analogue (ex: 362 nm, em: 520 nm) was measured before and 5 min after the addition of 2.3 μM rPGAM1 protein to the reaction mixture. Decrease in fluorescence intensity of 2,3-BPG analogue indicates 2,3-BPG analogue binding to rPGAM1 protein. The values are presented as relative fluorescence units (RFU). ( c ) Purified Flag-PGAM1 WT or Y26F were incubated with cofactor (represented by 2,3-BPG analogue, 8-hydroxy-1,3,6-pyrenetrisulfonate). The cofactor binding affinity was determined by decrease in fluorescence intensity of the analogue. The values are presented as RFU. The error bars represent mean values±s.d. from three independent experiments (*0.01< P <0.05; ** P <0.01). Full size image To test this hypothesis, we incubated active rFGFR1 with purified, recombinant PGAM1 WT and Y26F mutant in an in vitro kinase assay, followed by incubation with a competitive 2,3-BPG fluorescent analogue (8-hydroxy-1,3,6-pyrenetrisulfonate) [18] , [19] ( Fig. 2b ). The decrease in fluorescence (ex: 362 nm, em: 520 nm) compared with buffer control was measured as 2,3-BPG binding ability. Phosphorylation of PGAM1 WT by FGFR1 resulted in a significant increase in the amount of bound 2,3-BPG analogue, whereas substitution of PGAM1 Y26 abolished enhanced binding of cofactor in the presence of rFGFR1 ( Fig. 2c ). Moreover, a quantitative mass spectrometry-based study ( Fig. 3a ) revealed that the H11 phosphorylation levels of Y26F mutant is significantly lower compared with PGAM1 WT in an in vitro kinase assay using PGAM1 proteins incubated with rFGFR1 in the presence of 2,3-BPG ( Fig. 3b ). Similar results were obtained when using Flag-tagged mouse PGAM1 (mPGAM1) WT and Y26F from ‘rescue’ H1299 cells with stable knockdown of endogenous human PGAM1 (hPGAM1) and rescue expression of Flag-mPGAM1 WT or Y26F mutant, respectively ( Fig. 3d ). These results suggest that Y26 phosphorylation may enhance PGAM1 activity by stabilising the H11-phosphorylated PGAM1. 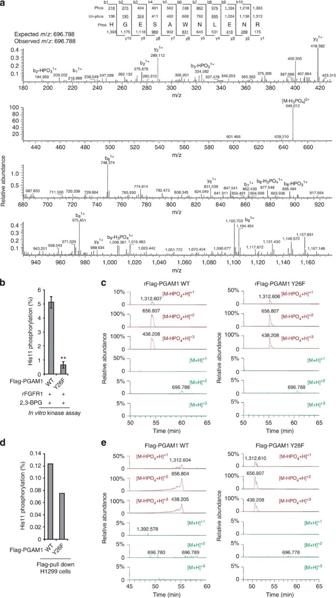Figure 3:Y26 phosphorylation results in increased H11 phosphorylation of PGAM1in vitroandin vivo. (a) Detection of H11 phosphorylation in PGAM1 using LC-MS/MS. Tandem mass spectrometry (MS/MS) spectrum of phosphorylated PGAM1 peptide pHGESAWNLENR (residue number 11–21) collected using collision-induced dissociation (CID) fragmentation. Underlined nominal masses above and below the sequence denote the b and y ions, respectively that were annotated from the spectrum. The expected and observed mass to charge ratio (m/z) for the [M+2H+]2+precursor ion is provided. [M-H3PO4]+2 represents molecular ion with loss of the phosphate group. (b,c) Phosphorylation by rFGFR1 leads to increased H11 phosphorylation of Flag-PGAM1 WT but not Y26F in the presence of 10 μM 2,3-BPG (b). Panel (c) shows relative quantification of H11-phosphorylated PGAM1 using reverse phase liquid chromatography. MS data for HGESAWNLENR (upper three red spectra in each panel) and pHGESAWNLENR (lower three green spectra in each panel) were used to calculate the relative levels of phosphorylated and unphosphorylated peptide across all observable charge states in Flag-tagged PGAM1 WT and Y26F mutant incubated with active FGFR1 and 2,3-BPG for one hour (c, left and right, respectively). The relative abundance was normalised to the largest peak of each scan, which corresponds to 5.5E7 (c, left) and 2.26E7 (c, right). (d,e) Rescue cells expressing mouse PGAM1 (mPGAM1) Y26F demonstrate reduced H11-phosphorylated levels compared with cells with mPGAM1 WT (d). WT or Y26F: cells with stable knockdown of endogenous hPGAM1 and rescue expression of mPGAM1 WT or Y26F mutant, respectively. Panel (e) shows relative quantification of H11-phosporylated PGAM1 using reverse phase liquid chromatography with Flag-tagged PGAM1 WT and Y26F mutant proteins isolated from rescue H1299 cells (e, left and right, respectively). The relative abundance was normalised to the largest peak of each scan, which corresponds to 1.12E7 (e, left) and 1.96E7 (e, right). The error bars represent mean values±s.d. from two independent experiments (*0.01<P<0.05; **P<0.01). Figure 3: Y26 phosphorylation results in increased H11 phosphorylation of PGAM1 in vitro and in vivo . ( a ) Detection of H11 phosphorylation in PGAM1 using LC-MS/MS. Tandem mass spectrometry (MS/MS) spectrum of phosphorylated PGAM1 peptide pHGESAWNLENR (residue number 11–21) collected using collision-induced dissociation (CID) fragmentation. Underlined nominal masses above and below the sequence denote the b and y ions, respectively that were annotated from the spectrum. The expected and observed mass to charge ratio (m/z) for the [M+2H + ] 2+ precursor ion is provided. [M-H3PO4]+2 represents molecular ion with loss of the phosphate group. ( b , c ) Phosphorylation by rFGFR1 leads to increased H11 phosphorylation of Flag-PGAM1 WT but not Y26F in the presence of 10 μM 2,3-BPG ( b ). Panel ( c ) shows relative quantification of H11-phosphorylated PGAM1 using reverse phase liquid chromatography. MS data for HGESAWNLENR (upper three red spectra in each panel) and pHGESAWNLENR (lower three green spectra in each panel) were used to calculate the relative levels of phosphorylated and unphosphorylated peptide across all observable charge states in Flag-tagged PGAM1 WT and Y26F mutant incubated with active FGFR1 and 2,3-BPG for one hour ( c , left and right, respectively). The relative abundance was normalised to the largest peak of each scan, which corresponds to 5.5E7 ( c , left) and 2.26E7 ( c , right). ( d , e ) Rescue cells expressing mouse PGAM1 (mPGAM1) Y26F demonstrate reduced H11-phosphorylated levels compared with cells with mPGAM1 WT ( d ). WT or Y26F: cells with stable knockdown of endogenous hPGAM1 and rescue expression of mPGAM1 WT or Y26F mutant, respectively. Panel ( e ) shows relative quantification of H11-phosporylated PGAM1 using reverse phase liquid chromatography with Flag-tagged PGAM1 WT and Y26F mutant proteins isolated from rescue H1299 cells ( e , left and right, respectively). The relative abundance was normalised to the largest peak of each scan, which corresponds to 1.12E7 ( e , left) and 1.96E7 ( e , right). The error bars represent mean values±s.d. from two independent experiments (*0.01< P <0.05; ** P <0.01). Full size image Y26 phosphorylation stabilises H11-phosphorylated PGAM1 To further understand the structural properties of Y26-phosphorylation-enhanced activation of H11-phosphorylated PGAM1, we crystalised human PGAM1 with phosphorylated H11 (1.65 Å; Supplementary Table S1 ) from purified PGAM1 protein incubated with 2,3-BPG, in which the occupancy of phosphate on H11 was refined to be 0.70; mass spectrometry analysis of the 2,3-BPG-treated PGAM1 supports that the majority of PGAM1 protein was phosphorylated ( Supplementary Fig. S1a ). We also crystalised the apo-form of non-phosphorylated WT human PGAM1 (2.08 Å) as previously reported [16] . Both structures of the H11-phosphorylated and non-phosphorylated forms were superposed with a RMSD value of 0.34 Å ( Supplementary Fig. S1b ). Upon comparison between these two structures, we found a major conformational change at the loop 12–23 in the H11-phosphorylated form, which is close to H11 that is in the active site of PGAM1 ( Fig. 4a ). Further structural analysis revealed that, in the structure of non-phosphorylated PGAM1 form, Y26 docks on W16 in the flexible loop ( Fig. 4b ), while the negative charged E19 is located in the positively charged active site, blocking access of cofactor (2,3-BPG) and substrate (3-PG) to the active site ( Fig. 4c ). Moreover, E19 forms hydrogen bonds with residues S14 and S23 on the loop, which stabilise the conformation of non-phosphorylated PGAM1 ( Fig. 4c ). In contrast, Y26 is exposed to the surface in the structure of the H11-phosphorylated form of PGAM1, whereas E19 flips away from the active site to allow the negatively charged phosphate group of phosphorylated H11 to be accommodated ( Fig. 4d ). In addition, the phosphorylated-H11 forms extensive hydrogen bonds with adjacent residues, including R10, R62, E89, H186 and G187, through its phosphate group ( Fig. 4d ). These hydrogen bonds also contribute to the stabilisation of the phosphorylated-histidine group captured in the crystal, which, otherwise, is generally unstable in the aqueous solution with a half-life around 30 min (ref. 20 ). 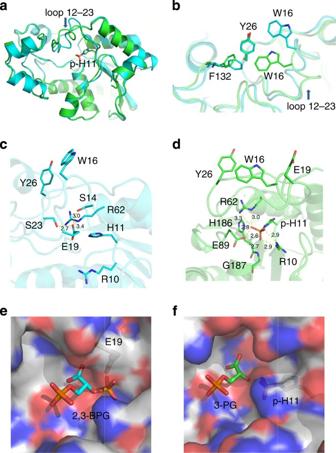Figure 4: Y26 phosphorylation may release E19 from blocking the active site of PGAM1. (a) Superposition of PGAM1 WT (cyan) and H11-phosphorylated form (green). Phosphorylated H11 is shown in stick and loop 12–23 with the large conformational change is marked. (b) Comparison of Y26 surrounding residues between WT PGAM1 (cyan) and H11-phosphorylated form (green). (c) Interactions between E19 and adjacent residues in Y26 buried WT PGAM1. (d) Interactions between phosphorylated H11 and adjacent residues in Y26 exposed phosphorylated PGAM1. (e) Superposed cofactor 2,3-BPG in the active site of non-phosphorylated PGAM1. There is a clash between E19 and phosphate group of 2,3-BPG. (f) Superposed substrate 3-PG in active site of H11-phosphorylated PGAM1 showing that it is ready to react with phosphorylated H11. Figure 4: Y26 phosphorylation may release E19 from blocking the active site of PGAM1. ( a ) Superposition of PGAM1 WT (cyan) and H11-phosphorylated form (green). Phosphorylated H11 is shown in stick and loop 12–23 with the large conformational change is marked. ( b ) Comparison of Y26 surrounding residues between WT PGAM1 (cyan) and H11-phosphorylated form (green). ( c ) Interactions between E19 and adjacent residues in Y26 buried WT PGAM1. ( d ) Interactions between phosphorylated H11 and adjacent residues in Y26 exposed phosphorylated PGAM1. ( e ) Superposed cofactor 2,3-BPG in the active site of non-phosphorylated PGAM1. There is a clash between E19 and phosphate group of 2,3-BPG. ( f ) Superposed substrate 3-PG in active site of H11-phosphorylated PGAM1 showing that it is ready to react with phosphorylated H11. Full size image These data together suggest a model in which Y26 phosphorylation may shift the protein conformation to release the negatively charged E19 that blocks the active site ( Fig. 4e ), thus promoting 2,3-BPG binding and consequently H11 phosphorylation, which may also help to keep the active site open for substrate (3-PG) binding ( Fig. 4f ). Please see below for detailed discussion. Y26 Phosphorylation of PGAM1 is common in human cancer cells We also generated an antibody that specifically recognises PGAM1 phospho-Y26 ( Supplementary Fig. S2a ). We found that PGAM1 is commonly expressed and phosphorylated at Y26 in diverse leukaemia and multiple myeloma cells associated with various constitutively activated tyrosine kinase mutants, as well as various human solid tumour cells including lung, prostate, breast and head and neck cancer cells ( Fig. 5a ). In addition, we found that PGAM1 protein expression and Y26 phosphorylation levels are upregulated in primary leukaemia cells from diverse acute myeloid leukaemia, chronic myelogenous leukaemia and B-cell acute lymphoblastic leukaemia patients ( n =5), compared with control peripheral blood cells from healthy donors ( n =4) ( Supplementary Fig. S2b ), and PGAM1 protein levels are significantly upregulated in head and neck tumour samples compared with normal tissue controls detected by immunohistochemical staining ( Supplementary Fig. S2c ). In in vitro kinase assays, purified PGAM1 proteins were directly phosphorylated at Y26 by diverse recombinant, active oncogenic tyrosine kinases including FGFR1, EGFR, FLT3 and JAK2 ( Fig. 5b ). Moreover, inhibiting FGFR1 by treatment with TKI258 resulted in decreased PGAM1 Y26 phosphorylation in FGFR1-expressing lung cancer H1299 cells and leukaemia KG-1a cells ( Fig. 5c ; left and right, respectively). In addition, inhibition of FLT3-ITD by TKI258 ( Fig. 5d ) and JAK2 by AG490 ( Fig. 5e ) resulted in decreased Y26 phosphorylation of PGAM1 in the pertinent human cancer cell lines. 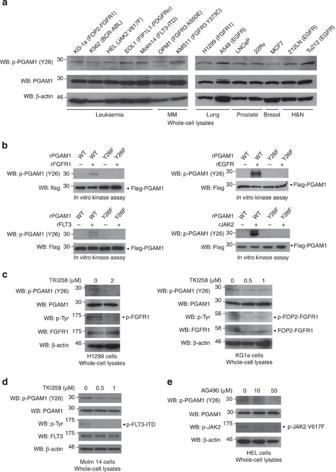Figure 5: Y26 phosphorylation is common in diverse cancer cells. (a) Protein expression and Y26 phosphorylation levels of PGAM1 in diverse human leukaemia, multiple myeloma (MM), lung, prostate, breast, and head and neck (H and N) cancer cells were assessed by western blot. Oncogenic tyrosine kinases associated with individual cancer cells are indicated. (b) Y26 phosphorylation levels of rPGAM1 incubated with active, recombinant rFGFR1, rEGFR, FLT3 (rFLT3) or JAK2 (rJAK2) in diversein vitrokinase assay were detected by western blot. (c–e) Immunoblotting results showing Y26 phosphorylation levels of PGAM1 in lung cancer H1299 (c; left) and leukaemia KG-1a (c: right) cells upon treatment with FGFR1 inhibitor TKI258, in leukaemia Molm14 cells (associated with FLT3-ITD mutant) treated with TKI258 (d), and leukaemia HEL cells (associated with JAK2 V617F mutant) treated with JAK2 inhibitor AG490 (e). Figure 5: Y26 phosphorylation is common in diverse cancer cells. ( a ) Protein expression and Y26 phosphorylation levels of PGAM1 in diverse human leukaemia, multiple myeloma (MM), lung, prostate, breast, and head and neck (H and N) cancer cells were assessed by western blot. Oncogenic tyrosine kinases associated with individual cancer cells are indicated. ( b ) Y26 phosphorylation levels of rPGAM1 incubated with active, recombinant rFGFR1, rEGFR, FLT3 (rFLT3) or JAK2 (rJAK2) in diverse in vitro kinase assay were detected by western blot. ( c – e ) Immunoblotting results showing Y26 phosphorylation levels of PGAM1 in lung cancer H1299 ( c ; left) and leukaemia KG-1a ( c : right) cells upon treatment with FGFR1 inhibitor TKI258, in leukaemia Molm14 cells (associated with FLT3-ITD mutant) treated with TKI258 ( d ), and leukaemia HEL cells (associated with JAK2 V617F mutant) treated with JAK2 inhibitor AG490 ( e ). Full size image Y26 phosphorylation of PGAM1 promotes tumour growth In order to determine the role of Y26 phosphorylation of PGAM1 in cancer cell metabolism and tumour growth, we next generated ‘rescue’ H1299 cells as described [14] by RNAi-mediated stable knockdown of endogenous hPGAM1 and rescue expression of Flag-tagged mPGAM1 WT or Y26F ( Fig. 6a ). We found that, compared with mPGAM1 WT rescue cells, expression of the catalytically less active Y26F mutant attenuates PGAM1 activity in the presence of 2,3-BPG ( Fig. 6b ), which results in decreased glycolytic rate ( Fig. 6c ), oxidative PPP flux and NADPH/NADP + ratio ( Fig. 6d , respectively), as well as reduced anabolic biosynthesis including RNA and lipid biosynthesis using 14 C-glucose as carbon source, accompanied by reduced NADPH/NADP + ratio ( Fig. 6f , respectively). However, attenuation of PGAM1 by stable knockdown or expression of Y26F mutant does not affect lipid and RNA biosynthesis from 14 C-glutamine ( Supplementary Fig. S2d,e , respectively). Interestingly, attenuation of PGAM1 in cancer cells does not affect the intracellular ATP levels ( Fig. 6h ) or O 2 consumption rate ( Supplementary Fig. S2f ), nor sensitivity of cells to treatment with oligomycin, a mitochondrial ATP synthase inhibitor, with regard to ATP levels and O 2 consumption rate ( Fig. 6h and Supplementary Fig. S2f , respectively). These results together suggest that Y26 phosphorylation levels of PGAM1 are important for coordination between glycolysis and PPP/biosynthesis using glucose but not glutamine as a carbon source, while attenuation of PGAM1 does not significantly affect intracellular ATP levels. 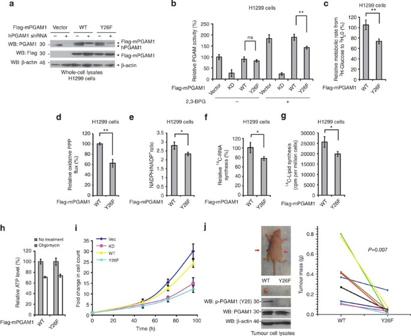Figure 6: Y26 phosphorylation of PGAM1 is important for glycolysis and anabolic biosynthesis as well as cell proliferation and tumour growth. (a) Generation of H1299 cells with stable knockdown of endogenous hPGAM1 and rescue expression of mPGAM1 WT or Y26F. (b) PGAM1 activity in rescue cells expressing mPGAM1 Y26F mutant was compared with that in control cells harbouring an empty vector or rescue cells expressing mPGAM1 WT, respectively, in the presence and absence of 2,3-BPG. (c–h) Glycolytic rate (c), oxidative PPP flux (d), NADPH/NADP+ratio (e), RNA biosynthesis (f), lipogenesis (g) and intracellular ATP levels in the presence or absence of 100 nM oligomycin (h) were measured in rescue cells expressing mPGAM1 Y26F mutant, compared with those in control rescue cells of mPGAM1 WT. (i,j) Rescue expression of catalytically less active Y26F mutant attenuates H1299 cell proliferation (i), as well as tumour growth potential of H1299 cells in xenograft nude mice (j). (j; left) Dissected tumours (indicated by red arrows) in a representative nude mouse; expression and Y26 phosphorylation levels of PGAM1 or mPGAM1 proteins in tumour lysates are shown. (j; right) Cells expressing mPGAM1 Y26F show significantly reduced tumour formation in xenograft nude mice compared with cells expressing mPGAM1 WT (P-values were determined by the paired Student’st-tests). The error bars represent mean values±s.d. from three independent experiments (*0.01<P<0.05; **P<0.01). Figure 6: Y26 phosphorylation of PGAM1 is important for glycolysis and anabolic biosynthesis as well as cell proliferation and tumour growth. ( a ) Generation of H1299 cells with stable knockdown of endogenous hPGAM1 and rescue expression of mPGAM1 WT or Y26F. ( b ) PGAM1 activity in rescue cells expressing mPGAM1 Y26F mutant was compared with that in control cells harbouring an empty vector or rescue cells expressing mPGAM1 WT, respectively, in the presence and absence of 2,3-BPG. ( c – h ) Glycolytic rate ( c ), oxidative PPP flux ( d ), NADPH/NADP + ratio ( e ), RNA biosynthesis ( f ), lipogenesis ( g ) and intracellular ATP levels in the presence or absence of 100 nM oligomycin ( h ) were measured in rescue cells expressing mPGAM1 Y26F mutant, compared with those in control rescue cells of mPGAM1 WT. ( i , j ) Rescue expression of catalytically less active Y26F mutant attenuates H1299 cell proliferation ( i ), as well as tumour growth potential of H1299 cells in xenograft nude mice ( j ). ( j ; left) Dissected tumours (indicated by red arrows) in a representative nude mouse; expression and Y26 phosphorylation levels of PGAM1 or mPGAM1 proteins in tumour lysates are shown. ( j ; right) Cells expressing mPGAM1 Y26F show significantly reduced tumour formation in xenograft nude mice compared with cells expressing mPGAM1 WT ( P -values were determined by the paired Student’s t -tests). The error bars represent mean values±s.d. from three independent experiments (*0.01< P <0.05; ** P <0.01). Full size image In addition, we found that ‘rescue’ cells expressing mPGAM1 Y26F mutant demonstrate decreased cell proliferation compared with control cells expressing mPGAM1 WT ( Fig. 6i ). Moreover, we functionally validated these findings by performing xenograft experiments. Nude mice were injected with Flag-mPGAM1 WT rescue H1299 cells on the left flank and Y26F rescue cells on the right flank ( Fig. 6j ). Ten million cells of each cell line were injected and the mice were monitored for tumour growth over a 6-week time period. The masses of tumours derived from PGAM1 Y26F rescue cells were significantly reduced compared with those of tumours formed by Flag-mPGAM1 WT cells ( Fig. 6j ). Y26 phosphorylation of PGAM1 regulates 3-PG and 2-PG levels We recently reported that PGAM1 coordinates glycolysis and anabolic biosynthesis by controlling intracellular levels of its substrate 3-PG and product 2-PG, which consequently inhibits 6PGD in the oxidative PPP and activates 3-PHGDH in serine biosynthesis to provide feedback regulation of 3-PG levels, respectively [4] . In consonance with these findings, we found that, compared with the mPGAM1 WT rescue cells, rescue expression of the catalytically less active Y26F mutant results in increased 3-PG ( Fig. 7a ) and decreased 2-PG ( Fig. 7b ) levels, as well as reduced anabolic biosynthesis of RNA and lipids ( Fig. 7c , respectively) and decreased cell proliferation ( Fig. 7e ), while treatment with a cell permeable form of 2-PG (methyl-2-PG) significantly rescues these phenotypes. These data together suggest that PGAM1 Y26 phosphorylation levels, in addition to PGAM1 protein expression levels [4] , are also important to control intracellular 3-PG and 2-PG levels, which confers both metabolic and proliferative advantages to cancer cells. 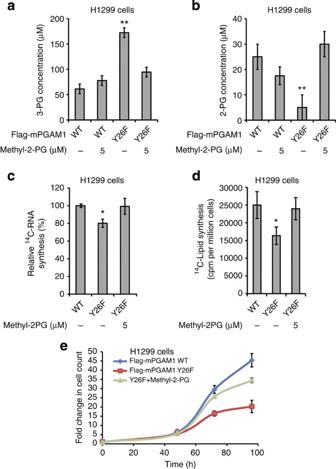Figure 7: Y26 phosphorylation of PGAM1 controls 3-PG and 2-PG levels to regulate biosynthesis and proliferation. (a–e) Intracellular 3-PG (a) and 2-PG levels (b), RNA biosynthesis (c), lipogenesis (d) and cell proliferation rate (e) in H1299 cells expressing mPGAM1 Y26F mutant were measured, compared with control cells with rescue expression of mPGAM1 WT, in the presence and absence of cell permeable methyl-2-PG. The error bars represent mean values±s.d. from three independent experiments (*0.01<P<0.05; **P<0.01). Figure 7: Y26 phosphorylation of PGAM1 controls 3-PG and 2-PG levels to regulate biosynthesis and proliferation. ( a – e ) Intracellular 3-PG ( a ) and 2-PG levels ( b ), RNA biosynthesis ( c ), lipogenesis ( d ) and cell proliferation rate ( e ) in H1299 cells expressing mPGAM1 Y26F mutant were measured, compared with control cells with rescue expression of mPGAM1 WT, in the presence and absence of cell permeable methyl-2-PG. The error bars represent mean values±s.d. from three independent experiments (*0.01< P <0.05; ** P <0.01). Full size image Upregulated expression of PGAM1, likely due to loss of TP53 , has been demonstrated in diverse human tumours and leukaemias [4] , [9] , [10] . In the current report, our findings suggest that, besides the commonly increased gene expression of PGAM1 that is likely due to loss of p53 in cancer cells, Y26 phosphorylation represents an alternative molecular mechanism underlying PGAM1 upregulation in human cancers. Y26 phosphorylation of PGAM1 is common in diverse human cancers and has been detected in a number of phospho-proteomics studies performed by our collaborators at Cell Signalling Technology Inc. using a spectrum of human cancer cells and primary tissue samples from human cancer patients ( http://www.phosphosite.org/siteAction.do?id=11589 ). As tyrosine kinase signalling is commonly upregulated in human cancers, our findings suggest that phosphorylation of Y26 enhances PGAM1 activity, which may represent a common, short-term molecular mechanism underlying upregulated PGAM1 activity in both leukaemias and solid tumours, in addition to the chronic upregulation of PGAM1 gene expression that is believed to be due to loss of TP53 in cancer cells. Moreover, our findings that Y26 phosphorylation could stabilise the active conformation of PGAM1 suggest a novel mechanism by which PGAM1 activity is regulated. Our structural analyses suggest that Y26 phosphorylation could shift the PGAM1 conformation that releases the negatively charged E19 from blocking the active site. By docking 2,3-BPG to the active site of PGAM1 based on a previously published crystal structure of bisphosphoglycerate mutase in complex with 2,3-BPG ( Fig. 4e ) [21] , we observed that E19 blocks the active site of the protein and consequently prevents binding of the cofactor 2,3-BPG, which is required to transfer a phosphate group to H11, leading to H11 phosphorylation. As we obtained H11-phosphorylated PGAM1 crystal by incubating purified, recombinant PGAM1 protein with excess 2,3-BPG, it is likely that PGAM1 can be ‘phosphorylated’ by 2,3-BPG at H11 in the absence of Y26 phosphorylation. This also explains the results presented in Fig. 1d–g , which show that phosphorylation of PGAM1 by FGFR1 serves only to enhance PGAM1 activation in the presence of 2,3-BPG. However, our structural data suggest that activation of PGAM1 would benefit from a conformational change that precludes Y26 from forming hydrophobic interactions with W16. This is accomplished when Y26 is phosphorylated and thus negatively charged, which leads to exposure of Y26 to the surface. This further stabilises the active, H11-phosphorylated conformation, in which E19, a residue that blocks the active site of the non-phosphorylated protein ( Fig. 4e ), moves away to accommodate 2,3-BG binding and consequently allow H11 phosphorylation. Moreover, the active site with exposed Y26 in the H11-phosphorylated PGAM1 is more accessible for the substrate 3-PG ( Fig. 4f ), and such a conformation is further stabilised by the multiple hydrogen bonds formed between phosphorylated H11 and its surrounding residues ( Fig. 4d ). The relatively low H11 phosphorylation quantified by MS using recombinant protein or cell lysates can be attributed to the fact that histidine phosphorylation is usually very unstable. In the protein (MALDI-MS and crystal) the phospho-H11 is stabilised with surrounding residues of phospho-H11 that contribute to its stability. Upon digestion to peptide, the stabilization effect of the protein is lost and the phosphorylated histidine is unstable with a half-life of 35 min. The fact that we observed H11 phosphorylation in the protein crystal structure strongly indicates the protein-mediated stabilization of this typically quite labile modification. Therefore, our findings suggest that Y26 phosphorylation can shift the protein conformation that contributes to PGAM1 activation and further stabilise the active form of PGAM1. Furthermore, our findings for the first time elucidate the structural mechanism by which H11 phosphorylation contributes to PGAM1 activation. Phospho-H11 activates PGAM1 at least in part, by promoting substrate 3-PG binding. Recently, Vander Heiden et al . [22] showed that the pyruvate kinase substrate, phosphoenolpyruvate (PEP) can transfer a phosphate to PGAM1 to ‘phosphorylate’ the catalytic H11 on PGAM1, producing pyruvate in the absence of PKM2 activity. We tested this concept and found that FGFR1-dependent enhancement of PGAM1 activity is not altered in the presence of physiological levels of PEP (30 μM) ( Supplementary Fig. S3 ). This suggests that Y26 phosphorylation- and PEP-dependent H11 phosphorylation are independent mechanisms that contribute to PGAM1 activation. We recently reported that PGAM1 regulates anabolic biosynthesis by controlling intracellular levels of its substrate 3-PG and product 2-PG (ref. 4 ). The concentrations of these glycolytic metabolites can directly affect the catalytic activity of enzymes involved in PPP (3-PG binds to and inhibits 6PGD in the oxidative PPP) and biosynthesis (2-PG activates PHGDH in serine biosynthesis pathway), which represents a novel, additional link between glycolysis, PPP and biosynthesis. Inhibition of PGAM1 by shRNA or a small molecule inhibitor PGMI-004A results in increased 3-PG and decreased 2-PG levels in cancer cells, leading to significantly decreased glycolysis, PPP flux and biosynthesis, and reduced cancer cell proliferation and tumour growth [4] . In consonance with these findings, substitution of Y26 attenuates PGAM1 activity, leading to accumulation of 3-PG and reduction of 2-PG in cancer cells, accompanied by decreased glycolysis, PPP/anabolic biosynthesis and cell proliferation, as well as tumour growth in xenograft mice. It is somewhat surprising that treatment with 5 μM methyl-2-PG rescues the decreased 2-PG level to ~30 μM in cells expressing PGAM1 Y26F mutant. We hypothesize that upon treatment, cell permeable methyl-2-PG enters the cell via passive diffusion, moving down its concentration gradient from outside the cell (5 μM) to inside the cell (0 μM). Once inside the cell, methyl-2-PG is hydrolysed to 2-PG, which is not cell permeable and chemically different from methyl-2-PG. Thus, the conversion of methyl-2-PG to 2-PG eliminates intracellular methyl-2-PG, which sustains the concentration gradient of methyl-2-PG across the cell membrane (extracellular 5 μM versus intracellular 0 μM). This in turn facilitates continuous diffusion of methyl-2-PG into cells, and if the diffusion and hydrolysis of methyl-2-PG occur more quickly than 2-PG consumption in glycolysis, restoration of physiological 2-PG levels (~30 μM) inside the cells could be eventually achieved. Together, these data suggest that Y26 phosphorylation may provide a regulatory window for cancer cells to promptly respond to changes of nutrients and microenvironment, at least in part by altering intracellular levels of 3-PG and 2-PG to coordinate glycolysis and biosynthesis, providing a metabolic advantage to cancer cell proliferation and tumour growth. Mass spectrometry analysis Determination of histidine phosphorylation was performed using reversed phase high pressure liquid chromatography-mass spectrometry. The immunoprecipitated beads were washed with TBS and Flag-tagged PGAM1 proteins were eluted by 3 × FLAG peptide in TBS (Sigma) and directly subjected to MS analysis. PGAM1 WT and Y26F mutant samples were resolved using SDS–PAGE, and PGAM1 containing bands were excised. Bands were digested with trypsin (Promega) overnight at 25 °C, and tryptic peptides were extracted with repeated desiccation and swelling in acetonitrile and 100 mM ammonium bicarbonate, respectively. The extracted peptides were concentrated by vacuum centrifugation and desalted using in-house made C18STAGE Tips before mass spectrometric analysis. Samples were loaded by an Eksigent AS2 autosampler onto a 75-μm fused silica capillary column packed with 11 cm of C18 reverse phase resin (5 μm particles, 200 Å pore size; Magic C18; Michrom BioResources). Peptides were resolved on a 110-min 1–100% buffer B gradient (buffer A=0.1 mol l −1 acetic acid, Buffer B=70% acetonitrile in 0.1 mol l −1 acetic acid) at a flow rate of 200 ml min −1 (1200 series; Agilent). The HPLC was coupled to a mass spectrometer (LTQ-Orbitrap; ThermoFisher Scientific) with a resolution of 30,000 for full MS followed by seven data-dependent MS/MS analyses. Collision-induced dissociation was used for peptide fragmentation. Targeted runs were also performed to increase the likelihood of quantifying the labile histidine phosphorylation. Peptide abundance of the phosphorylated and unphosphorylated peptides was calculated by manual chromatographic peak integration of full MS scans using Qual Browser software (version 2.0.7; ThermoFisher Scientific Inc.). The relative abundance of the phosphorylated peptide was calculated as the ratio of the sum of the areas underneath the peaks of phosphorylated peptide to the sum of the areas underneath peaks corresponding to phosphorylated and unphosphorylated peptides (total peptide). The peptide sequence and histidine phosphorylation were confirmed by manual inspection of the MS/MS spectra. Sample preparation of H11-phosphorylated PGAM1 protein Purified PGAM1 protein (100 μM, in 20 mM Tris-HCl buffer, pH 7.4) mixed with 2,3-BPG (final concentration: 500 μM) and incubated for half an hour at room temperature. Excess 2,3-BPG was removed by desalting. Purified protein and 2,3-BPG-treated protein were directly analysed by MALDI-TOF mass spectrum using sinapic acid as matrix solution. Crystallization of PGAM1 proteins and data collection Crystals of PGAM1 were originally identified using the PEG ION crystallization screen kit (Hampton Research). Optimised crystals were produced using hanging drop vapour diffusion at 16 °C by mixing 1 μl of protein solution at 30–40 mg ml −1 with 1 μl reservoir solution containing 0.1 M MES pH 6.0, 8% PEG 3350. Crystals appeared after 1 h and continued to grow for several days. Non-phosphorylated PGAM1 was obtained by eluting with 500 mM imidazole from the Ni-NTA column and storing the PGAM1 under 277 K for 1 week. The protein was then washed by with buffer A (10 mM Tris, pH8.0, 500 mM NaCl) containing 20% glycerol three times and then purified by gel filtration. Phosphorylated PGAM1 crystals were obtained by treating WT PGAM1 with 5 mM 2,3-BPG for half an hour and excess 2,3-BPG were removed by buffer exchange before crystallization. Crystals were dehydrated by 50% PEG 6,000 for 24 h, and quickly frozen in liquid nitrogen. All diffraction data were collected at 100 K at the macromolecular crystallography for life science beamline LS-CAT (21-ID-F) and NE-CAT (24-ID-C), respectively, at the Advanced Photon Source, Argonne National Laboratory. Native data sets extending to 1.65 Å resolution were collected at 0.9795 Å wavelength (12.66 keV). The data were processed with HKL2000 and the scaled data were used for molecular replacement. Crystallographic statistics are summarized in Supplementary Table S1 . Data refinement For phasing, model building and refinement, the structures of both PGAM1-apo form and phosphorylated PGAM1 were determined by molecular replacement using Phaser in the CCP4 suite, with the template protein as the search model (PDB accession code: 1YFK). The structures were then refined by using Phenix. Manual rebuilding of the model was carried out using the molecular graphics program COOT based on electron density interpretation. Water molecules were incorporated into the model if they gave rise to peaks exceeding 3σ in Fo-Fc density maps. The final refined models have good stereochemistry with 98.5% of the residues in the most favored regions of the Ramachandran plot with none in the disallowed regions (values calculated using PROCHECK from CCP4 suite). Xenograft studies Approval of use of mice and designed experiments was given by the Institutional Animal Care and Use Committee of Emory University. Nude mice (nu/nu, male 6–8-week old, Charles River Laboratories) were subcutaneously injected with 10 × 10 6 H1299 cells stably expressing mPGAM1 WT and Y26F with stable knockdown of endogenous hPGAM1 on the left and right flanks, respectively. Tumour growth was recorded by measurement of two perpendicular diameters of the tumours over a 6-week course using the formula 4π/3 × (width/2) 2 × (length/2). The tumours were harvested and weighed at the experimental endpoint, and the masses of tumours (g) derived from cells expressing mPGAM WT or Y26F mutant in both flanks of each mouse were compared. Statistical analyses have been done by comparison in relation to the control group with a two-tailed paired Student’s t -test. Accesssion codes: Coordinates and structure factors for PGAM1-apo and H11-phosphorylated PGAM1 have been deposited in the Protein Data Bank under accession codes 4GPI and 4GPZ , respectively. How to cite this article: Hitosugi, T. et al . Tyr26 phosphorylation of PGAM1 provides a metabolic advantage to tumours by stabilizing the active conformation. Nat. Commun. 4:1790 doi: 10.1038/ncomms2759 (2013).